Stimulated emission from nitrogen-vacancy centres in diamond Stimulated emission is the process fundamental to laser operation, thereby producing coherent photon output. Despite negatively charged nitrogen-vacancy (NV − ) centres being discussed as a potential laser medium since the 1980s, there have been no definitive observations of stimulated emission from ensembles of NV − to date. Here we show both theoretical and experimental evidence for stimulated emission from NV − using light in the phonon sidebands around 700 nm. Furthermore, we show the transition from stimulated emission to photoionization as the stimulating laser wavelength is reduced from 700 to 620 nm. While lasing at the zero-phonon line is suppressed by ionization, our results open the possibility of diamond lasers based on NV − centres, tuneable over the phonon sideband. This broadens the applications of NV − magnetometers from single centre nanoscale sensors to a new generation of ultra-precise ensemble laser sensors, which exploit the contrast and signal amplification of a lasing system. The negatively charged nitrogen-vacancy centre in diamond [1] has found wide applicability in quantum information [2] , [3] , [4] and sensing [5] of magnetic fields [6] , [7] , [8] , [9] , [10] , [11] , electric fields [12] , [13] , temperature [14] , [15] , pressure [16] and biosensing [17] , [18] . For both readout and sensing, fluorescence that is, spontaneous emission is collected and the spin state is inferred from the different emission levels. The time-averaged spontaneous emission from the different spin states differs by no more than 30% and spontaneous emission is in all directions, creating the challenge of collecting the emission [19] . Photons created by stimulated emission, on the other hand, have the same phase, wavelength and spatial mode as the stimulating light field. This enables close-to-unity collection efficiency as all photons are emitted into the same mode. Furthermore, the competition between spontaneous emission and stimulated emission potentially allows contrast of several orders of magnitude between the brightest and least bright state of the NV − centre compared with the typical 30% for single centres and 4% for ensembles under spontaneous emission. Stimulated emission is also the basis for lasing, but despite the success of diamond Raman lasers [20] and despite an early proposal for a laser based on diamond defects [21] , and the demonstration of cavity coupling [10] , [22] a realization of an NV laser has not been demonstrated so far. Microscopy, based on stimulated emission depletion, a super-resolution technique taking advantage of emission reduction by a strong light field, has been successfully implemented with NV centres [23] as well as NVN centres [24] . However, the photophysical process leading to said emission reduction, be it stimulated emission to the ground state, or photo-ionization to the charge neutral NV 0 state [25] , [26] , [27] has not been extensively studied in this context. Indeed, photo-ionization of the NV − ↔NV 0 has been shown to be induced by strong light pulses [28] , [29] , [30] , [31] . The ionization process has been suggested to be a two-photon process [26] , [28] , [29] , which scales quadratically with laser power, for the wavelengths around the zero-phonon line (ZPL) of NV emission. Excited state absorption, for example via the ionization channel, can lead to weakening of stimulated emission by driving towards NV 0 . Insight into stimulated emission of NV centres is particularly important, since both ionization and stimulated emission by a strong light pulse result in reduced NV − spontaneous emission and are therefore hard to distinguish, and also owing to the multitude of applications benefiting from these competing processes. Here we show experimentally that light with wavelengths above 650 nm does not induce net ionization of NV − centres, for powers up to a few Watts during the pulse, and show strong evidence for the presence of stimulated emission in the NV − phonon side band. We use a green (532 nm) CW pump-laser together with a pulsed laser source with tunable wavelength to measure stimulated emission at different wavelengths. The pulses, with a duration of only 6 ps, provide an intense light field and create a measurable change in the emission properties. Since the emitted photons are indistinguishable from the laser pulse, we initially detect the stimulated emission indirectly by the reduction of spontaneous emission. In subsequent measurements, we demonstrate enhanced emission at the wavelength of the stimulating laser as direct evidence for stimulated emission. In addition, we measure the excited state population of both charge states separately by monitoring the corresponding ZPL intensities to detect any potential ionization. Our results show the presence of stimulated emission and the possibility of lasing with NV − centres. Stimulated emission and experimental setup Conventionally, both sensing and quantum state readout in the NV − centre is performed via fluorescence measurements after optical pumping, typically by exciting at a wavelength around 532 nm, from the 3 A 2 ground state, which we denote |1〉, to the 3 E excited state |2〉, see Fig. 1a . Spontaneous emission occurs at a rate ≈(12 ns) −1 over the characteristic NV − spectrum with ZPL at 637 nm, corresponding to the |1〉↔|2〉 transition, and with phonon-sideband emission from 637 to ∼ 800 nm, corresponding to transitions from |2〉 to short-lived vibronic states slightly above |1〉 with added phonons, followed by a rapid decay to |1〉 (refs 32 , 33 ). 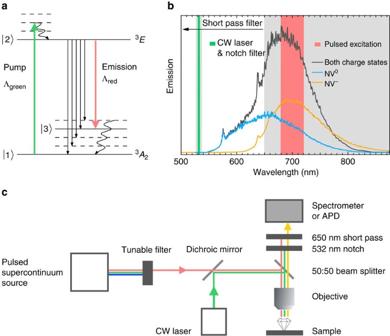Figure 1: Stimulated emission and experimental setup. (a) Nitrogen-vacancy centre (NV−) level structure including phonon-added states (dashed and |3〉) with pumping and emission rates. Laser pumping (green) lifts population to the excited state, which can then decay via spontaneous emission (straight black arrows) or stimulated emission (red) due to interaction with a light field whose wavelength matches the |2〉↔|3〉 transition. (b) Laser excitation (red and green columns) with short pass and notch (grey). This setup blocks laser light from the detector but still allows to monitor both NV−and NV0emission. Example spectra are included: NV−emission (orange), NV0emission (blue) and mixed emission (grey). (c) Experimental setup. Figure 1: Stimulated emission and experimental setup. ( a ) Nitrogen-vacancy centre (NV − ) level structure including phonon-added states (dashed and |3〉) with pumping and emission rates. Laser pumping (green) lifts population to the excited state, which can then decay via spontaneous emission (straight black arrows) or stimulated emission (red) due to interaction with a light field whose wavelength matches the |2〉↔|3〉 transition. ( b ) Laser excitation (red and green columns) with short pass and notch (grey). This setup blocks laser light from the detector but still allows to monitor both NV − and NV 0 emission. Example spectra are included: NV − emission (orange), NV 0 emission (blue) and mixed emission (grey). ( c ) Experimental setup. Full size image Stimulated emission due to a coherent light field of wavelength λ interacting with the NV centre occurs at a rate Λ red = σ λ I /( ħω λ ) where I is the power per area of the light field, ħω λ the corresponding photon energy and σ λ the stimulated emission cross-section, which as a function of λ is proportional to the NV emission spectrum, that is, the spontaneous emission rate. Strong stimulated emission is achieved by strong fields, produced for example, in optical cavities or in our case by a pulsed supercontinuum source. The rate of stimulated emission is increased for laser light in the phonon-sidebands’ wavelengths because the phonon-sideband emission is stronger than the ZPL emission, therefore the cross-section for decay on the phononic sidebands is higher. Accordingly, we choose a pulsed laser excitation around 700 nm (red light) at the peak of the phonon sideband, Fig. 1b , to achieve strong stimulated emission at the same wavelength. This laser is resonant with the transition between the excited state |2〉 and a phonon-added ground state |3〉 and induces a stimulated emission rate, which competes with the spontaneous emission, Fig. 1a . The red laser will therefore enhance the emission probability around 700 nm and reduce the emission probability for the rest of the NV spectrum. For lasing, population inversion is also easier to obtain on the sideband transition since the population in |3〉 decays quickly and therefore it is no longer necessary to pump more than 50% of the NV centres out of the ground state |1〉. Our present setup, however, is not designed for self-sustained lasing because the light field does not build up in a cavity but is provided by the pulsed laser. The stimulated emission can therefore not be measured directly, since it is indistinguishable from the stronger pulsed laser signal. However the reduction in the rest of the NV emission spectrum can be detected. This reduction can be turned on and off with the red laser. Obtaining full NV emission spectra is challenging when a strong laser at the centre of the NV emission spectrum ( ∼ 700 nm) is used. We used a 650 nm short pass and a 532 nm notch in front of the detector to block out the pulsed red laser and the green (532 nm) CW pump laser respectively before the light was detected with a spectrometer or avalanche photodiode detector (APD), Fig. 1b . This detection window allowed us to monitor both the NV − ZPL at 637 nm as well as the NV 0 ZPL at 575 nm. Ionization is expected to increase the emission of one peak at the cost of the other and can be clearly distinguished in this setup from stimulated emission, which should decrease the emission in the entire monitored range of wavelengths. Even in the case that ionization NV − ↔NV 0 occurs both ways during the 6 ps pulse, the emission spectrum, which is mainly obtained in the 12.5 ns between pulses, should reflect the new relative charge state populations. The short pass optical filter allows us to vary the red laser wavelength, that is, measure stimulated emission as a function of wavelength. We used a pulsed supercontinuum source (Fianium WL SC400-8) with a 6 ps pulse duration at a repetition rate of up to 80 MHz with a tunable filter, Fig. 1c , which allowed us to select both the centre wavelength (700 nm initially) and bandwidth (40 nm initially). The resulting time-averaged power of several mW corresponds to several Watts, during the pulse duration. The pulsed light was aligned via a dichroic mirror with the green CW laser and focused through an objective (NA=0.9) onto the NV diamond samples. We confirmed the effects on two ∼ 500 μm thick single-crystal diamonds as well as a nanodiamond sample, all with very high NV density. Emission reduction of both ZPLs To investigate the effect of the pulsed laser on the spontanteous emission, we first measured the NV emission between 550 and 650 nm when only the green CW laser excites the sample. We then measured the spectra when both the green CW and the pulsed laser at 700 with 40 nm bandwidth are on. The data in Fig. 2a was taken over 100 ms acquisition time, which corresponds to 8 million pulses. The spectra are integrated over the entire acquisition time including the pulsed laser being on and off, and the spectra were smoothed with a running average over a 4 nm window. 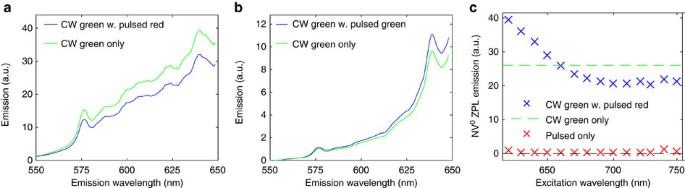Figure 2: Emission reduction of both zero-phonon lines. (a) Spectral emission of the NV centre ensemble due to 532 nm continuous wave (CW) laser excitation alone (green), and due to an added pulsed 700 nm laser excitation (blue). The emission with both lasers on is reduced compared with only green CW excitation. This is consistent with a preferential emission at 700 nm due to stimulated emission. (b) When the pulsed laser wavelength is changed to also be at 532 nm, the emission is increased by the pulsed laser. All the spectra were smoothed with a 4 nm window. (c) Two regimes exist: the NV0emission is decreased by the addition of pulsed laser wavelengths above 680 nm, where stimulated emission dominates, and increased for pulsed wavelengths below 640 nm, where ionization from NV−to NV0is known to be the dominant process. In the measured range of wavelengths the pulsed laser alone does not create any NV0signal, that is, there is no direct excitation. The pulsed power was kept constant at 2.9 mW for all excitation wavelengths. Figure 2a shows the emission with both the NV 0 ZPL at 575 nm and NV − ZPL at 637 nm clearly visible as expected since 532 nm pumping is known to excite both charge states of the NV. More importantly, the addition of the red pulsed laser reduces the entire emission in the observed wavelengths as expected when stimulated emission at 700 nm is induced. We note that the reduction occurs despite the fact that the red pulsed laser by itself creates weak excitation of the NV − as discussed later. Both ZPLs (NV − and NV 0 ) are reduced, which indicates that the reduction of NV − emission is not caused by ionization towards NV 0 . If ionization to NV 0 occurred, then we would expect the increased NV 0 population to provide an increase of the NV 0 ZPL emission. Quite contrary, in Fig. 2a the NV 0 ZPL is also reduced indicating that the NV 0 population also experiences stimulated emission at 700 nm. While this might seem surprising, the phonon sideband of the NV 0 extends over a slightly wider range than the NV − and is quite strong at 700 nm, see Fig. 1b . Figure 2: Emission reduction of both zero-phonon lines. ( a ) Spectral emission of the NV centre ensemble due to 532 nm continuous wave (CW) laser excitation alone (green), and due to an added pulsed 700 nm laser excitation (blue). The emission with both lasers on is reduced compared with only green CW excitation. This is consistent with a preferential emission at 700 nm due to stimulated emission. ( b ) When the pulsed laser wavelength is changed to also be at 532 nm, the emission is increased by the pulsed laser. All the spectra were smoothed with a 4 nm window. ( c ) Two regimes exist: the NV 0 emission is decreased by the addition of pulsed laser wavelengths above 680 nm, where stimulated emission dominates, and increased for pulsed wavelengths below 640 nm, where ionization from NV − to NV 0 is known to be the dominant process. In the measured range of wavelengths the pulsed laser alone does not create any NV 0 signal, that is, there is no direct excitation. The pulsed power was kept constant at 2.9 mW for all excitation wavelengths. Full size image Our interpretation attributes the emission reduction in the observed wavelength range to stimulated emission at 700 nm. As an initial check of this interpretation, we changed the pulsed laser wavelength to also be 532 nm, as the CW source. This is outside the NV emission spectrum and stimulated emission should therefore not occur. Figure 2b shows that in this case indeed the addition of the pulsed laser increases the total emission, proving that the effect of emission reduction by the added pulsed laser only occurs at certain wavelengths. For stimulated emission, this range of wavelengths would be expected to be the range of spontaneous emission, which we confirm further below. How can the apparent occurrence of stimulated emission be brought into agreement with the established fact [25] , [26] , [27] , [28] , [29] , [30] , [31] that strong light pulses around 637 nm efficiently decharge the NV − to the NV 0 ? To explore the photoionization, we reduced the pulsed laser wavelength, swapping the 650 nm short pass for a 600 nm short pass and monitored the NV 0 ZPL. Again, we combined a green CW laser, which creates NV 0 emission, with the pulsed red light, which by itself does not create NV 0 emission. Any change in the NV 0 signal after adding pulsed light must therefore be due to either stimulated emission or ionization. Figure 2c shows clearly the transition between two regimes: For pulsed light at high wavelengths, λ >680 nm, the NV 0 signal is reduced as discussed above and stimulated emission dominates. For pulsed light at lower wavelengths, λ <640 nm, the NV 0 signal is increased and ionization from NV − towards the NV 0 is the dominant process [25] . The threshold between the two behaviours seems to be around 660 nm, that is, a photon energy of 1.88 eV. This energy value is slightly higher than theoretical calculations of the minimal energy value required for ionization from the NV − excited state, which were predicted as 1.56 eV in ref. 29 and 1.7 eV (private communication with Audrius Alkauskas). Note that this value is not to be confused with the ionization energy from the NV − ground state of 2.6 eV (ref. 28 ). The relative emission reduction at the NV − ZPL in Fig. 2a is about 18% and about 21% in the measurement of Fig. 2c for 700 nm pulsed wavelength. Assuming that the red intensity in the region of focus is intense enough to fully deplete the excited state via stimulated emission, this means that 18 to 21% of the NV centres that contribute to the signal are in the region of focus. Since we used a 500 μm thick sample, the percentage value of focus volume relative to illuminated volume seems high but is realistic given that there is non-uniform intensity in all dimensions of the laser spot and considering that NV centres in the focus volume contribute more strongly to the emission signal. Emission dynamics While stimulated emission should only occur during the 6 ps pulse duration, a reduction by other indirect effects could show other timescales or no temporal structure. Changes in the emission due to ionization have been found to occur typically on much slower timescales of microseconds to milliseconds [25] , [26] , [30] . We therefore measured the total emission (not spectrally resolved) in the detected emission window (550 nm to 650 nm, see Fig. 1b ) with an APD and time-correlated counting card with a 0.1 ns temporal resolution. While the 6 ps pulse is not resolved on that scale, the dynamics between pulses is resolved. The time between pulses was set to 25 ns, corresponding to a repetition rate of 40 MHz. 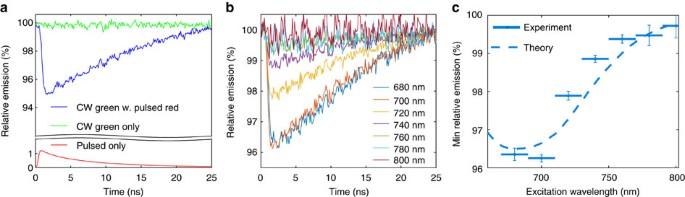Figure 3: Temporal emission reduction for different stimulating wavelengths. (a): raw data of temporally resolved emission which is spectrally integrated below 650 nm. The fluorescence reduction occurs instantly at the point in time of the red pulse. Then the emission recovers in between pulses. (b) Temporal emission curves for different pulsed excitation wavelengths (c) The minimal relative emission directly after the pulse as a function of the pulsed excitation wavelength shows that the greatest reduction in emission occurs around 700 nm corresponding to the peak of the phonon sideband of the NV. The error bars give the standard deviation of the temporal data points averaged for each value. Figure 3a shows that the reduction due to the added pulsed laser (blue curve) relative to the green CW laser (green curve) occurs faster than the time resolution of the electronics and then the signal recovers between pulses due to the green CW pump, as expected. The emission due to the pulsed laser only (red curve) shows that the 700 nm pulse alone actually weakly excites the NV − centre. The time point of this excitation coincides with the reduction of the emission of the blue curve, that is, the time point of the pulse. Figure 3: Temporal emission reduction for different stimulating wavelengths. ( a ): raw data of temporally resolved emission which is spectrally integrated below 650 nm. The fluorescence reduction occurs instantly at the point in time of the red pulse. Then the emission recovers in between pulses. ( b ) Temporal emission curves for different pulsed excitation wavelengths ( c ) The minimal relative emission directly after the pulse as a function of the pulsed excitation wavelength shows that the greatest reduction in emission occurs around 700 nm corresponding to the peak of the phonon sideband of the NV. The error bars give the standard deviation of the temporal data points averaged for each value. Full size image To further investigate the wavelength dependence, discovered in Fig. 2 , we varied the centre wavelength of the pulsed laser in 20 nm steps. The full width at half maximum of the laser was also set to 20 nm to ensure no overlap between the steps. The strength of the reduction varies with the wavelength of the pulsed laser ( Fig. 3b,c ) and shows that the effect is the strongest at 700 nm and reduces towards 800 nm. To ensure the data are independent of the small power variations of the source, which occurred when changing wavelengths, we measured the power for each wavelength and rescaled the reduction accordingly. Figure 3c shows the relative emission level right after the pulse (averaged over 10 data points). As expected for stimulated emission, the effect occurs for wavelengths within the NV emission spectrum and is strongest around 700 nm, which corresponds to the peak of the phonon sideband. To understand the temporal dynamics, we modelled the NV by a simple three-state system ( Fig. 1a ). This model neglects the spin dynamics but is a good approximation since the green CW laser spin-polarizes into the m s =0 state and all emission processes are spin-conserving. The differential equations for the system probabilities P j to be in the states | j 〉 in Fig. 1a are: where the pulsed laser created a stimulated emission rate Λ red ( t ) with a temporal Gaussian profile with standard deviation 6 ps, repetition rate of (25 ns) −1 =40 MHz and overall strength is fitted to match the experiment. When we give time-independent values for Λ red below, we give the equivalent rate that a 6 ps square pulse would have. The spontaneous emission rate to |3〉 was taken to be L 23 =18 MHz from ref. 34 . All spontaneous emission rates to states other than |3〉 were grouped into one rate of L 21 =65.3 MHz directly from state |2〉 to state |1〉. The value was chosen to correspond to a total lifetime of 12 ns for the excited state. The phonon-decay rate was set to L 31 =1 THz but the exact value is irrelevant provided it is fast compared to all other transition rates. Starting the system in state |1〉 with the constant pumping rate Λ green we time-evolved the system via numerical integration until it reached a steady state; we then included the time-dependent repeating red pulses in the evolution. In the simulations without the red pulses, the steady state has a given population in the excited state. Including the red pulses leads to stimulated emission on the |2〉 to |3〉 transition over the 6 ps pulse duration. This depletes population from the excited state to |3〉, which then decays to |1〉 due to the fast phononic decay. In the 25 ns between the pulses, the population of the excited state slowly recovers to its original value due to the constant green pumping rate. The number of spontaneously emitted photons also drops during the pulse duration and then recovers in between pulses because it is proportional to the excited state population. The timescale of the recovery is roughly the time between pulses, that is, 25 ns, and decreases (that is, the recovery rate increases) with increasing green CW pump power. To quantify the expected wavelength dependence for the effect for stimulated emission, we modelled different wavelengths of the pulsed laser by varying the stimulated emission cross section proportional to the measured NV emission spectrum with a maximum of Λ red =6 GHz at 682 nm. The pump rate was set to Λ green =92 MHz and Fig. 3c shows that the resulting theoretical wavelength dependence of the relative emission matches qualitatively with the experimental measurements. We note that a transition rate of order GHz is realistic for a pulsed source with powers of few W during the 6 ps pulse, and a focus-area on the order 1 μm 2 . The wavelength dependence is further evidence for stimulated emission as opposed to ionization. Ionization of the NV centre has been explained as an absorption process from the excited state to the conduction band. The absorption to the conduction band should therefore not show any wavelength dependence since the band can accommodate different photon energies. There should only be a sharp drop of the effect once the photon energy becomes too small (that is, wavelength too long) to reach the conduction band. Ionization should furthermore be more likely with increased excited state population, that is, increased absorption. If the emission reduction was caused by ionization then the wavelength dependence would follow the absorption spectrum of the NV, which has its phonon sideband and maximum in wavelength range around 550 nm (below the ZPL) and not around 700 nm (above the ZPL) [25] . While the pulsed laser wavelength changes the strength of the emission reduction, it does not seem to change the timescale of the recovery in Fig. 3b . This behaviour matches our simulations. The recovery of the emission in between pulses is approximately exponential. In the case that the effect is caused by stimulated emission the recovery should be purely caused by the green CW pump. For other effects, such as ionization, the recovery could be either explained with the crystal returning to its equilibrium state, with a rate set by internal NV or crystal parameters, which should be slower and independent of the green pump rate. For ionization, the recovery could also be explained by the green laser ionizing back to the NV − state, which has previously been measured to occur at a rate of (0.25 μs) −1 for a 532 nm laser at 0.25 mW power (see Fig. 3c in ref. 26 ), which is an order of magnitude slower than the rate we find. 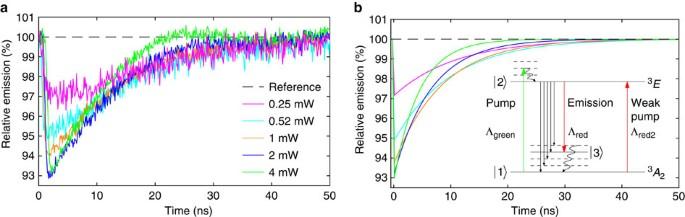Figure 4: Emission reduction and recovery for different green CW powers. (a) Experimental data where the red pulse was att≈1 ns. The recovery rate increases with increasing green power. The time-averaged red power was measured as 1.73 mW. (b) The theoretical modelling, reproducinga. Figure 4a shows a measurement of the emission dynamics with varying powers of the green CW pump power. The pulse repetition rate was reduced to (100 ns) −1 =10 MHz to ensure that the system has enough time to return to its equilibrium state between pulses. Since stronger green CW pumping leads to higher total emission, we plot the relative emission as a percentage of the highest total emission respectively. We observed a shorter recovery time, i.e., faster recovery rate, for stronger green CW power: in Fig. 4a , the lowest power (pink curve) has the slowest recovery rate. With increasing green power (light blue, orange, dark blue), the emission recovers faster and the highest power (green) shows the fastest recovery rate. The recovery time for 0.25 mW (pink) is ∼ 25 ns, which is much faster than the expected 250 ns for ionization [26] . The recovery timescales are consistent with stimulated emission as demonstrated below. For lower green powers, the relative emission reduces to only ∼ 97% (pink) rather than ∼ 93% (green and dark blue). This is explained by the fact that the red pulsed laser weakly excites the NV as demonstrated below. Figure 4: Emission reduction and recovery for different green CW powers. ( a ) Experimental data where the red pulse was at t ≈1 ns. The recovery rate increases with increasing green power. The time-averaged red power was measured as 1.73 mW. ( b ) The theoretical modelling, reproducing a . Full size image The observed dynamics was reproduced by our simulations: corresponding curves are plotted in the same colours in Fig. 4a,b . The stimulated emission rate was set to Λ red =13 GHz to reproduce the relative emission reduction to ∼ 93% for large powers. The pump rates were varied proportional to the green laser powers in the experiment from 8.8 to 141 MHz, which corresponds to an average focus area of (0.6 μm) 2 , given the known absorption cross-section 0.95 × 10 −16 cm 2 (ref. 35 ). These pump rates lead to recovery timescales similar to the experiment both in absolute values and relative trend between the curves. To reproduce the fact that lower green powers show a weaker emission reduction effect, we included an excitation rate of Λ red2 =0.85 GHz due to the red pulse from ground to excited state: This rate Λ red2 was calculated using the weak effective absorption cross-section for NV − at 700 nm, which we measured to be 3 × 10 −2 m 24 . We had initially neglected this as it is only a weak effect but we found that for low green powers (which resulted in weak total emission) the inclusion of this effect in the modelling was a good explanation for why the pink curve only reduces to ∼ 97% while higher green powers reduce to ∼ 93%. All measurements so far were taken with single crystal diamond. We compared a single crystal sample to nanodiamonds on a silicon substrate under the same conditions. The same effects were observed and confirmed the generality of our results, see Supplementary Note 1 . Direct measurement of stimulated emission As final confirmation that the emission reduction is caused by stimulated emission we have measured the stimulated emission at the stimulating wavelength directly. To measure the stimulated emission signal against the much stronger red laser signal and its associated noise, we have modulated the green pump laser with a frequency of 548 Hz and changed the red laser from a pulsed to a CW source. For details of the setup, see Fig. 5a and the ‘Methods’ section. Thus, a stimulated emission signal due to the green pump laser must also be modulated, while the red laser signal is not. A lock-in amplifier allowed us to filter only the frequency of interest and thus removed the red laser signal and a majority of the noise. 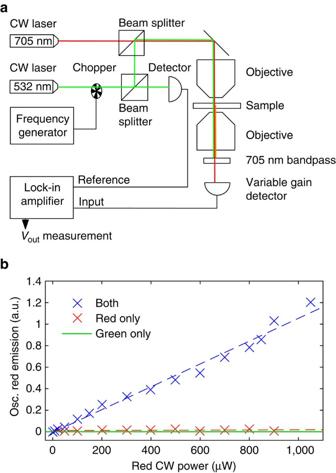Figure 5: Direct measurement of stimulated emission. (a) Setup with modulation on the green laser and a lock-in amplifier filtering the detection signal for only the modulation frequency (b) The red CW laser creates stimulated emission. Because the stimulated emission is dependent on the green pump laser, it also oscillates at the modulation frequency and is hence detected. The red CW laser signal itself is unmodulated and is thus filtered out by the lock-in amplifier. The green laser by itself creates fluorescence, which is almost entirely filtered out by the 705 nm bandpass and additionally only the fraction that is emitted into the solid angle of the objective is directed to the detector. The stimulated emission is emitted into the laser beam direction and is thus entirely collected by the detector and gives a clear signal linear with stimulating power. The blue and red dashed lines are linear fits. Figure 5b shows that the resulting signal is indeed almost zero when only the red CW laser is on. When only the modulated green pump is on some spontaneous emission is produced at the modulation frequency but we block most of that out with a 705 nm bandpass filter to see only stimulated emission. When the red CW laser is added to the green pump laser, Fig. 5 shows that the emission signal increases linearly with the red stimulating laser power. This increase is only measured because it oscillates at the modulation frequency of the green pump and is thus clearly stimulated emission because it is pumped with the green laser and emitted due to the red laser. This is the first direct measurement of stimulated emission from the NV centre. We note that the spontaneous emission signal from only the green laser is negligible compared with the stimulated emission signal for two reasons: We used a bandpass filter around the red laser wavelength and thus removed the majority of spontaneous emission and additionally the spontaneous emission is isotropic and only the fraction of the solid angle of the collecting objective is detected whereas the stimulated emission is directional in the stimulating beam direction and therefore has very high collection efficiency. This leads to the given configuration with excellent contrast between the stimulated emission signal and the spontaneous emission from the green laser. For higher green powers, the spontaneous emission signal strengthens while the detection contrast is not as strong. This measurement was performed in transmission through the sample using an objective on each side, see Fig. 5a . Figure 5: Direct measurement of stimulated emission. ( a ) Setup with modulation on the green laser and a lock-in amplifier filtering the detection signal for only the modulation frequency ( b ) The red CW laser creates stimulated emission. Because the stimulated emission is dependent on the green pump laser, it also oscillates at the modulation frequency and is hence detected. The red CW laser signal itself is unmodulated and is thus filtered out by the lock-in amplifier. The green laser by itself creates fluorescence, which is almost entirely filtered out by the 705 nm bandpass and additionally only the fraction that is emitted into the solid angle of the objective is directed to the detector. The stimulated emission is emitted into the laser beam direction and is thus entirely collected by the detector and gives a clear signal linear with stimulating power. The blue and red dashed lines are linear fits. Full size image We have shown clear signatures of stimulated emission in NV centres in single crystal diamond as well as nanodiamonds. We demonstrated the spontaneous NV emission from a green CW pump laser and the reduction of this spontaneous emission due to a strong pulsed red laser at the centre of the phonon sideband ( ∼ 700 nm). We explain this reduction in spontaneous emission as being due to stimulated emission at 700 nm. The measured emission reduction follows all the expected behaviour for stimulated emission in terms of its dependence on the wavelength of the pulsed laser, the spectral reduction of both the NV − and the NV 0 ZPL, as well as the temporal dynamics, including emission reduction during the laser pulse and a recovery rate that varies with the green laser power. Our theoretical modelling of stimulated emission also reproduces the measured effects. Particularly we show that for wavelengths ∼ 700 nm stimulated emission is the dominant process over ionization. This is indicated by no increase of either ZPL line, a wavelength dependence, which follows the emission rather than the absorption spectrum and a temporal dynamics inconsistent with ionization. We furthermore showed the transition to the regime where ionization dominates, which is when the pulsed laser is set to wavelengths around the NV − ZPL. Our results are therefore consistent with previously reported photoionization studies NV − ↔NV 0 induced by wavelengths below 650 nm. Our findings manifest that stimulated emission dominating over ionization is dependent on the wavelength (rather than the intensity), which should be in the phonon sideband λ >650 nm. This is in agreement with previous literature on super-resolution microscopy, where stimulated emission depletion was achieved with wavelengths λ >700 nm pulses [36] , [37] , [38] , whereas charge state depletion was achieved with 637 nm pulses [39] , [40] . The measurement of the effect in both single-crystal diamond and nanodiamonds shows sample-independent applicability. Our results show that stimulated emission can be utilized in the NV and lead the way to exploring the benefits of stimulated emission, for example, for higher collection efficiency into a cavity mode. Our results also indicate that NV centres are suitable as a laser medium. This opens up new avenues of applications for the NV centre. We estimate the conditions for lasing with NV centres for the three-phonon sideband transition at 709 nm, where stimulated emission strongly dominates. Lasing is possible, when the rate of stimulated emission into an optical cavity is greater than the loss rate κ of the cavity. The stimulated emission rate can be calculated [41] , [42] on the basis of the cavity and spontaneous emission characteristics. From this condition, we find the minimum density of NV centres to achieve lasing: where c is the speed of light, n =2.4 the refractive index of diamond, λ =709 nm the free-space wavelength of the three-phonon sideband, ν 23 = c / λ the corresponding frequency, Δ ν 23 ≈24 THz the corresponding width of the three-phonon peak [15] , [43] , l cav the cavity length, the cavity finesse, V cav the cavity mode volume and V diam the diamond volume within the cavity mode. From this equation, we see that the required density reduces proportional to 1/finesse and that lasing is in principle possible with a commonly achieved density of 0.1 to 1 p.p.m. even for low-finesse cavities. However, low-finesse cavities will require very large pump powers for lasing. The required power at the lasing threshold can be estimated by the absorption cross-section and enforcing the detailed balance condition for the excited and ground state population ρ exc / ρ gr =Γ/Λ with pumping rate Λ and emission rate Γ at threshold, which is valid for not too small NV numbers in the cavity. We obtain This shows that while lasing is challenging, it should be possible, for example, for a cavity of 1 mm length with finesse =10 5 and average illumination area A cav =1 mm 2 and an illuminated diamond volume that is half the cavity volume with an NV concentration [NV]=1 p.p.m. requiring a pump power of 240 mW. We confirmed numerically that this analytical approximation gives a good estimate for the required power by solving numerically the full seven-state model [1] of the NV centre coupled to a laser cavity [42] . Laser threshold magnetometry [42] was recently proposed as a novel way of measuring magnetic fields with NV centre ensembles, enabling higher contrast and stronger output signals using stimulated emission. By driving an NV laser at the threshold, sensitivities down to fT Hz −1/2 could be achieved and could enable a robust, room-temperature alternative for SQUID sensors. The current results support the feasibility of the laser threshold sensing scheme. Diamond sample preparation We confirmed the effects on different diamond samples: sample A was a single crystal, type 1b, irradiated with 2 MeV electrons to 2 × 10 18 e cm −2 , annealed at 800 °C for 5 h. Sample B was a single crystal, type 1b, irradiated with 2 MeV electrons to a fluence of 1.1 × 10 18 e cm −2 and annealed in vacuum at 900 °C for 2 h. During irradiation, the sample was in a dry nitrogen environment and kept at temperature below 800 °C to avoid any surface degradation. Sample C was a single crystal, type 1b, irradiated with 2 MeV electrons to a fluence of 1 × 10 18 e cm −2 and annealed in vacuum at 800 °C for 2 h. Sample C was 50 μm thin used specifically for Fig. 5 to fit between the two objectives. Sample D were nanodiamonds, see Supplementary Note 1 ,irradiated with 2 MeV electrons to a fluence of 1 × 10 18 e cm −2 , vacuum annealed at 800 °C for 2 h, then oxydized in air at 510 °C for 4 h. Lasing conditions calculations To obtain an analytical estimate for the required pump power P thresh , connected to the pump rate Λ thresh = P thresh σ /( A cav ħω ) via the known absorption cross-section σ and the photon energy ħω , we enforced the detailed balance, that is, the ratio of transition rates equal the ratio of populations for the ground and excited state ρ exc / ρ gr =Γ/Λ from which we obtain the excited state population ρ exc =Λ/(Γ+Λ)≈Λ/Γ for a high enough number of NV centres such that at threshold, which we confirmed numerically for . Combining the detailed balance condition with the lasing condition Gρ exc = κ for the coupling G of NV centres and cavity and cavity loss rate κ , we find the required pump rate for lasing Λ thresh =Γ κ / G from which we can then calculate the required power P thresh . We note that the expression becomes invalid when the absorbed power under homogeneous illumination P abs = n NV n C V cav Λ ħω > P thresh , since the laser medium becomes strongly absorbing in this case. Here n C is the carbon density of diamond. This can be easily monitored and happens for very long cavity designs and very high NV densities. Setup for direct measurement of stimulated emission For the direct measurement of stimulated emission, we modulated the green 532 nm laser with an optical chopper at a frequency of 548 Hz and combined this via a fibre beam splitter with a CW 705 nm red laser. Since the stimulated emission is directional in the stimulating beam direction, we measured in transition using one objective ( × 10, NA=0.25) to focus the beam inside the sample and one objective ( × 40 NA=0.65) to collect the light after passing the sample once. Owing to the short working distance of the lenses, we used a thin sample of only 50 μm thickness to ensure the ability to focus both objectives to the same point in the sample and collimate the outgoing beam. The signal was detected via a variable gain detector and then frequency filtered with a lock-in amplifier using the chopper frequency as a reference. Thus we ensured that only emission caused by the green pump laser was detected. Since the spontaneous emission is isotropic only the fraction that goes into the solid angle of the collecting lens is detected. The directional stimulated emission is collected entirely when the outcoming laser beam is collimated by the collecting objective. Data availability The data that support the findings of this study are available from the corresponding author on request. How to cite this article: Jeske, J. et al . Stimulated emission from nitrogen-vacancy centres in diamond. Nat. Commun. 8, 14000 doi: 10.1038/ncomms14000 (2017). Publisher's note: Springer Nature remains neutral with regard to jurisdictional claims in published maps and institutional affiliations.